Fractional quantum Hall effect in the absence of Landau levels It is well known that the topological phenomena with fractional excitations, the fractional quantum Hall effect, will emerge when electrons move in Landau levels. Here we show the theoretical discovery of the fractional quantum Hall effect in the absence of Landau levels in an interacting fermion model. The non-interacting part of our Hamiltonian is the recently proposed topologically non-trivial flat-band model on a checkerboard lattice. In the presence of nearest-neighbouring repulsion, we find that at 1/3 filling, the Fermi-liquid state is unstable towards the fractional quantum Hall effect. At 1/5 filling, however, a next-nearest-neighbouring repulsion is needed for the occurrence of the 1/5 fractional quantum Hall effect when nearest-neighbouring repulsion is not too strong. We demonstrate the characteristic features of these novel states and determine the corresponding phase diagram. As one of the most significant discoveries in modern condensed matter physics, fractional quantum Hall effect (FQHE) [1] has attracted intense theoretical and experimental studies in the past three decades. The wavefunctions proposed by Laughlin [2] , [3] , [4] first explained FQHE by introducing fractionally charged quasi-particles. Later, the ideas of flux attachment and the composite Fermi-liquid theory [5] have provided a rather simple but deep understanding of the nature of the FQHE. Among many of its interesting and unique properties, two of the most striking features of FQHE are the following: fractionalization, where quasi-particle excitations carry fractional quantum numbers and even fractional statistics of the constituent particles, and topological degeneracy, where the number of degenerate ground states responds non-trivially to the changing of the topology of the underlying manifold. These two phenomena are the central ideas of the topological ordering [6] . In addition, on the potential application side, they are also the essential components in the studies of topological quantum computation [7] . Since 1988, great efforts have been made to study quantum Hall effects in lattice models without Landau levels. The first such example is the theoretical model proposed by Haldane [8] , where it was demonstrated that in a half-filled honeycomb lattice, an integer quantum Hall state can be stabilized upon the introduction of imaginary hoppings. This study was brought to the forefront again recently owing to a major breakthrough in which a brand new class of topological states of matter, known as the time-reversal invariant Z 2 topological insulators, was discovered (see refs 9 , 10 and references therein). From the topological point of view, both Haldane's model and Z 2 topological insulators can be considered as generalizations of the integer quantum Hall effect. Unlike the FQHE, they do not support fractional excitations, and the ground states here have no topological degeneracy. For fractional states, fractional Z 2 topological insulators are found to be theoretically possible [11] . However, it is unclear how to realize such states with lattice models. This difficulty originates from the strong coupling nature of the fractionalized states. In contrast to the integer quantum Hall effect and the Z 2 topological insulators, where all their essential topological properties can be understood within a non-interacting picture, the interaction effects are expected to have a vital role in stabilizing a fractionalized topological state. In fact, without interactions, a fractional quantum Hall system will become a Fermi liquid due to the fractional filling factor. Most recently, a series of models with topologically non-trivial nearly flat-band models have been proposed [13] , [14] , [15] . These lattice models have topologically non-trivial bands (different from early proposal [16] ), similar to Haldane's model and Z 2 topological insulators, and their bandwidth can be tuned to be much smaller than the band gap, resulting in a nearly–flat-band structure. In particular, based on the mechanism of quadratic band touching [13] , [14] , a large class of flat-band models have been explicitly obtained with the ratio of the band gap to the bandwidth reaching the high value of 20–50. Owing to the strong analogy between these nearly flat bands and the Landau levels, it was conjectured that in these models, FQHE (or fractional topological insulators) can be stabilized in the presence of repulsive interactions. However, the conjecture is challenged by competing orders, for example, the charge-density wave, and thus the fate of these systems are unclear. More importantly, the flux attachment picture [5] may also break down, and it is very interesting to examine the nature of the corresponding emergent fractionalized quantum state, if it can be realized in such a model without Landau levels. Here we report the discovery of FQHE at filling factor 1/3 and 1/5 in models with topologically non-trivial nearly flat bands [14] , based on exact calculations of finite-size systems. The existence of the FQHE are confirmed by using two independent methods, both of which are well established and have been widely adopted in the study of the traditional FQHE. We have studied both the characteristic low-energy spectrum and the topologically invariant Chern numbers [17] , [18] , [19] , [20] , [21] , [22] of the low-energy states. The first method directly detects the topological degeneracy and the other is related to the phenomenon of fractionalization. Phase diagram We consider the following Hamiltonian on a checkerboard lattice: where H 0 describe the short-range hoppings in the two-band checkerboard-lattice model defined in ref. 14 , n i is the on-site fermion particle number operator. The nearest-neighbouring (NN) and next-nearest-neighbouring (NNN) bonds are represented by 〈 i , j 〉 and 〈〈 i , j 〉〉, respectively. 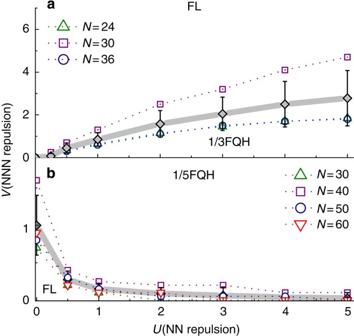Figure 1: Phase diagram for interacting flatband model. (a) At 1/3 and (b) 1/5 filling number in the parameter space of the nearest-neighbour (U) and next- nearest-neighbour (V) interaction strengths for different system sizes. In both (a) and (b), two phases are observed, the Fermi-liquid phase (labelled as FL) and the fractional-quantum-Hall phase (labelled as FQH). The dashed lines in both figures mark the phase boundaries at different system size. The thick grey lines mark the averaged phase boundary over different systems sizes and the error bar mark the averaged deviations. The effect of the NN ( U ) and NNN ( V ) interactions are summarized in the phase diagrams Figure 1a and b . At filling factor 1/3, the FQHE emerges by turning on a relatively small U . Interestingly, the FQHE phase remains robust at the large U limit, where particles avoid each other at NN sites and can only be destroyed by an intermediate V . At filling factor 1/5, the FQHE occurs in most region of the parameter space as long as the NNN repulsion V exceeds a critical value V c , whose value drops to zero for larger U . The observed FQHE states are characterized by nearly p -fold ( P =3 and 5 for filling factors 1/3 and 1/5 respectively) degenerating ground states with the momentum quantum numbers of these states related to each other by a unit momentum translation of each particle as an emergent symmetry, a finite spectrum gap separating the ground-state manifold (GSM) from the low-energy excited states with a magnitude dependent on the interaction strengths U and V , and the GSM carrying a unit total Chern number as a topological invariant protected by the spectrum gap, resulting in a fractional effect of 1/ p quantum for each energy level in the GSM. We identify the quantum phase transition on the basis of the spectrum-gap collapsing. As shown in Figure 1 , the Fermi-liquid phase with gapless excitations is found for relatively strong NNN interaction at 1/3 filling and for relatively weak NNN interaction at 1/5 filling. This observation is consistent with Haldane's pseudopotential theory [3] , and previous studies on ordinary FQHE, where a FQHE state is found to be sensitive to interactions and other microscopic details (for example, the thickness of the two-dimensional electron gas [23] ). Figure 1: Phase diagram for interacting flatband model. ( a ) At 1/3 and ( b ) 1/5 filling number in the parameter space of the nearest-neighbour ( U ) and next- nearest-neighbour ( V ) interaction strengths for different system sizes. In both ( a ) and ( b ), two phases are observed, the Fermi-liquid phase (labelled as FL) and the fractional-quantum-Hall phase (labelled as FQH). The dashed lines in both figures mark the phase boundaries at different system size. The thick grey lines mark the averaged phase boundary over different systems sizes and the error bar mark the averaged deviations. Full size image Low-energy spectrum and topological degeneracy Consider a system of N x × N y unit cells ( N s =2 N x N y sites) with twisted boundary conditions: , where T ( N j ) is the translation operator with j = x and y representing the x and y directions, respectively. Note that the filling factor is defined as the ratio of the number of particles ( N p ) over the number of unit cells ( N x × N y ). In the absence of impurities, the total momentum of the many-body state is a conserved quantity, and thus the Hamiltonian can be diagonalized in each momentum sector for systems with N s =24 to 60 sites (depending on filling factors). We consider periodic boundary conditions ( θ 1 = θ 2 =0) first. 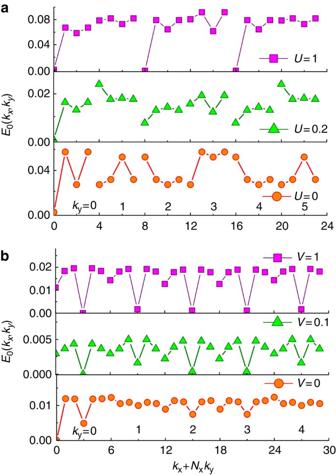Figure 2: Energy spectrum with interaction. (a) For 1/3 filling withV=0,U=0 to 1.0 (Uincreases from bottom panel up) andNs=2×4×6 sites; (b) For 1/5 filling withU=1 andV=0 toV=1 andNs=2×6×5. We have shifted the ground-state energy to zero for comparison. Nearly degenerate GSM and the large gap between GSM and excited states, observed in (a) at largeUand (b) at largeVindicate the formation of the fractional quantum Hall states. Figure 2a illustrates the evolution of the low-energy spectrum with changing U for V =0 and N s =2×4×6 ( N x =4 and N y =6) at particle-filling factor ν =1/3. Here the NN hopping strength ( t )is set to unity. We denote the momentum of a state q =(2 πk x / N x , 2 πk y / N y ) by using two integers ( k x , k y ) as shown in Figure 2 . For vanishing NN interaction U =0.0 (the bottom panel of Fig. 2a ), the ground state has k =(0,0) whereas no particular structure is observed in other k sectors. For a weak interaction U =0.2, we find an interesting change in the spectrum. Here the energies of two states with momenta ( k x , k y )=(0, 2) and (0, 4) have been lowered substantially. For a stronger interaction, the energies of the three states with k x =0 and k y =0, 2, 4 form a nearly degenerate GSM [6] at U >0.3. In the mean time, a sizable spectrum gap opens up, separating the GSM from the other excited states as shown in the top panel of Figure 2a for U =1.0. The obtained threefold ground state near degeneracy and a robust spectrum gap are the characteristic features of the 1/3 FQHE phase, which emerge with the onset of the NN repulsion U . By increasing the NNN repulsion V to a certain critical value V c , we have observed the collapse of the spectrum gap, which determines the boundary of the 1/3 FQHE phase, as shown in Figure 1a . 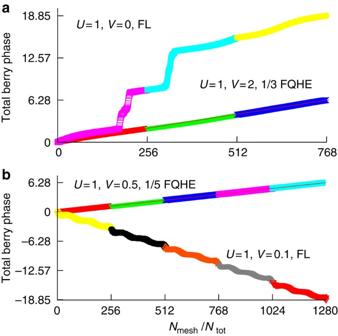Figure 3: Berry phase and topological quantization. The total Berry phase as a function ofNmesh/Ntot, which measures the ratio of the area in the boundary phase space for (a) 1/3 filling atNs=30; (b) 1/5 filling atNs=40. In fractional quantum Hall phase, a linear curve is observed whose slope is determined by filling factor, as expected. In the Fermi-liquid phase, we observed large fluctuation and non-universal behaviours, indicating the absence of the topological quantization. Further evidence of the FQHE based on topological quantization will be presented later in Figure 3 . Figure 2: Energy spectrum with interaction. ( a ) For 1/3 filling with V =0, U =0 to 1.0 ( U increases from bottom panel up) and N s =2×4×6 sites; ( b ) For 1/5 filling with U =1 and V =0 to V =1 and N s =2×6×5. We have shifted the ground-state energy to zero for comparison. Nearly degenerate GSM and the large gap between GSM and excited states, observed in ( a ) at large U and ( b ) at large V indicate the formation of the fractional quantum Hall states. Full size image Figure 3: Berry phase and topological quantization. The total Berry phase as a function of N mesh / N tot , which measures the ratio of the area in the boundary phase space for ( a ) 1/3 filling at N s =30; ( b ) 1/5 filling at N s =40. In fractional quantum Hall phase, a linear curve is observed whose slope is determined by filling factor, as expected. In the Fermi-liquid phase, we observed large fluctuation and non-universal behaviours, indicating the absence of the topological quantization. Full size image In Figure 2b , we present the formation of the 1/5 FQHE by showing the energy spectrum at particle filling factor ν =1/5 with increasing V at U =1 for a system with N s =2×6×5 ( N x =6 and N y =5). From the bottom panel to the top panel, five states with momenta (2, k y ) ( k y =0, ..., 4) form the nearly degenerate GSM with the increase of V , whereas a large spectrum gap is formed at V =1.0. The same feature of the energy spectrum is observed for the whole regime of the 1/5 FQHE above the critical V c line shown in the phase diagram Figure 1b while V c drops to near zero for larger U . We note that there is a small energy difference between the states in the GSM in both filling factors. This is a finite-size effect [21] , [24] as each of these states has to fit into the lattice structure. The finite-size effect is substantially smaller for 1/5 FQHE comparing with the 1/3 case due to the lower particle density. Interestingly, for all cases that we have checked for different system sizes ( N s =24–60), the members of the GSM are always related to each other through a momentum space translation as an emerging symmetry of the system. Namely, if ( k 1 , k 2 ) is the momentum quantum number for a state in the GSM, then another state in the GSM can be found in the momentum sector ( k 1 + N e , k 2 + N e ) modulo ( N x , N y ). This relation of the quantum numbers of the GSM demonstrates the correlation between the real space and momentum space in a manner precisely resembling the FQHE in a uniform magnetic field. For the case where the particle number N p is integer multiples of both N x and N y (for example, N s =2×3×6 and N s =2×5×5 at 1/3 and 1/5 fillings, respectively), all the states of the GSM are indeed observed to fall into the same momentum sector as expected. Fractional quantization of topological number To further establish the existence of the FQHE here, we study the topological property of the GSM by numerically inserting flux into the system using generalized boundary phases. As first realized by Thouless and co-workers [17] , [18] , [19] , a topological quantity of the wavefunction, known as the first Chern number, distinguishes the quantum Hall states from other topological trivial states. In particular, one can detect the fractionalization phenomenon in FQHE by examining the Chern number of the GSM through inserting flux into the system [20] , [21] , [22] . The results of this calculation are shown in Figure 3 . With details presented in the Methods part, the total Berry phase as a function of N mesh / N tot should be a linear function with slope 2 π /3 and 2 π /5 for the FQHE with filling factors 1/3 and 1/5, respectively. This agrees very well with the observation shown in Figure 3 . On the other hand, for the Fermi-liquid phase, strong fluctuations and non-universal behaviours of the Berry phase are found, suggesting the absence of topological quantization. FQHE at strong coupling limit We further examine the phase at strong coupling limit for lower filling factor ν =1/5, where 1/5 FQHE demonstrates less sensitivity to either large U or V . 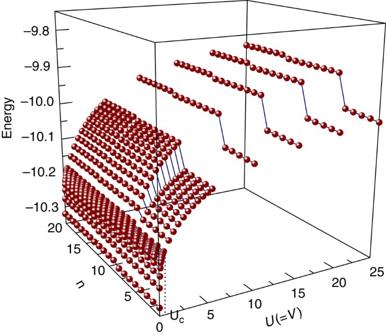Figure 4: Quantum phase transition and topological degeneracy. The low-energy spectrum for lowestnstates (n=1, ..., 20) as a function ofU(withV=U) for a system withNs=50. The dashed line marks the critical valueUc, at which the phase transition between a Fermi-liquid phase and the FQHE takes place. We show the lowest 20 eigenvalues as a function of U in Figure 4 , while we always set V = U for simplicity. At small U , we see the flatness of the spectrum in consistent with a Fermi-liquid phase with small energy dispersion. As we increase U > U c =0.35, all the lowest five states remain nearly degenerate, whereas higher energy states jump a step up making a robust gap between them and the GSM. In fact, the 1/5 FQHE persists into infinite U and V limit as we have checked by projecting out the configurations with double or more occupancy between a site and all its NN and NNN sites. Physically, this can be understood as particles at lower filling having enough phase space within the lower Hubbard band, and thus the FQHE remains intact. It would be very interesting to establish a variational state for the FQHE on the flatband model, which will be investigated in the future. Figure 4: Quantum phase transition and topological degeneracy. The low-energy spectrum for lowest n states ( n =1, ..., 20) as a function of U (with V = U ) for a system with N s =50. The dashed line marks the critical value U c , at which the phase transition between a Fermi-liquid phase and the FQHE takes place. Full size image Finally, it is important to emphasize that the fractional topological phases we found are very stable and the same effect survives even if the hopping strengths are tuned by an amount of ∼ 10%. On the experimental side, it is known that checker-board lattice we studied can be found in condensed matter systems (for example, the thin films of LiV 2 O 4 , MgTi 2 O 4 , Cd 2 Re 2 O 7 , etc. ), and the imaginary hopping terms we required can be induced by spin–orbit coupling and/or spontaneous symmetry breaking [25] . In addition, this lattice model also has the potential to be realized in optical lattice system using ultra-cold atomic gases, in which the tuning of the parameters are much easier compared with condensed matter systems. On the basis of these observations, we conclude that there is no fundamental challenge preventing the experimental realization of these novel fractional topological states, but further investigation is still needed to discover the best experimental candidates. Calculation of Chern number for many-body state The Chern number of a many-body state can be obtained as: where the closed path integral is along the boundary of a unit cell 0≤ θ ≤2 π with j = x and y , respectively. The Chern number C is also the Berry phase (in units of 2 π ) accumulated for such a state when the boundary phase evolves along the closed path. Equation (2) can also be reformulated as an area integral over the unit cell C =(1/2 π )∫ dθ 1 dθ 2 F , where F ( θ 1 , θ 2 ) is the Berry curvature. To determine the Chern number accurately [20] , [22] , we divide the boundary-phase unit cell into about N tot =200 to 900 meshe. The curvature F ( θ 1 , θ 2 ) is then given by the Berry phase of each mesh divided by the area of the mesh. The Chern number is obtained by summing up the Berry phases of all the meshes. Chern number quantization in FQHE We find that the curvature is in general a very smooth function of θ j inside FQHE regime. For an example, the ground-state total Berry phase sums up to 0.325×2 π , slightly away from the 1/3 quantization for a system with N s =30, U =1 and V =0 at 1/3 filling. Physically, as we start from one state with momentum ( k x , k y ) in the GSM, it evolves to another state with a different momentum k x → k x + N e ( k y → k y + N e ), when the boundary phase along x ( y ) direction is increased from 0 to 2 π . Thus, with the insertion of a flux, states evolve to each other within the GSM. We observe that only the total Berry phase of the GSM is precisely quantized to 2 π and the total Chern number C =1 for all different choices of parameters inside either the 1/3 or 1/5 FQHE regime of Figure 1 . When states in the GSM have the same momentum, the Chern number of each state is an integer due to non-crossing condition of the energy levels with the same quantum number, while the total Chern number remains the same [21] , [22] . Fluctuating Chern number in other phases As we move across the phase boundary from the FQHE state into the Fermi-liquid phase, there is no well-defined nearly degenerate GSM or spectrum gap, and the Berry curvature in general shows an order of magnitude bigger fluctuations. The obtained total Chern integer varies with system parameters (for example, U and V ). To illustrate this feature, we start from the lowest-energy eigenstate and continuously increase the boundary phases for three periods, which allows the first state to evolve into other states and eventually return back to itself. In Figure 3 , we plot the accumulated total Berry phase as a function of the ratio of the total meshes included N mesh over the total number of meshes N tot in each period. For the system in the 1/3 FQHE phase with N s =30, U =1 and V =0, the total Berry phase follows a straight line in all three periods, well fitted by , indicating a nearly perfect linear law of the Berry phase to the area in the phase space with a deviation around 10%. In the Fermi-liquid phase with N s =30, U =1 and V =2, we see step-like jumps of the total Berry phase, with a magnitude in the order of 2 π , in sharp contrast to the linear law in the FQHE phase. The total Chern number for the Fermi-liquid state sums up to three, indicating the decorrelation between three states. Different integer values for the Chern number are found in this region (including negative ones) with changing system parameters, demonstrating a measurable fluctuating Hall conductance if particles are charged. For 1/5 FQHE state, by following up the Berry phase of five periods for the ground state as shown in Figure 3b , we observe the same linear law with a slope of 2 π /5 and the total Chern number is quantized to one. Interestingly, a negative integer Chern number for Fermi-liquid state for the parameters U =1 and V =0.1 is observed confirming the non-universal nature of the topological number for such a gapless system. We conjecture that the Fermi-liquid phase may be unstable towards Anderson localization, especially at lower filling factors, similarly to the conventional FQHE systems [21] . How to cite this article : Sheng, D.N. et al . Fractional quantum Hall effect in the absence of Landau levels. Nat. Commun. 2:389 doi: 10.1038/ncomms1380 (2011).